TCTP directly regulates ATM activity to control genome stability and organ development inDrosophila melanogaster Translationally controlled tumour protein (TCTP) is implicated in growth regulation and cancer. Recently, human TCTP has been suggested to play a role in the DNA damage response by forming a complex with ataxia telangiectasia-mutated (ATM) kinase . However, the exact nature of this interaction and its roles in vivo remained unclear. Here, we utilize Drosophila as an animal model to study the nuclear function of Drosophila TCTP (dTCTP). dTCTP mutants show increased radiation sensitivity during development as well as strong genetic interaction with dATM mutations, resulting in severe defects in developmental timing, organ size and chromosome stability. We identify Drosophila ATM (dATM) as a direct binding partner of dTCTP and describe a mechanistic basis for dATM activation by dTCTP. Altogether, this study provides the first in vivo evidence for direct modulation of dATM activity by dTCTP in the control of genome stability and organ development. Protecting genome integrity from ionizing radiation (IR)-induced DNA damages is crucial for normal development and function of all organisms. To maintain genome integrity, cells perform a series of sophisticated and well-organized processes, termed the DNA damage response (DDR), which senses DNA lesions, transmits and amplifies this information to activate signalling cascades for DNA repair. Among various DNA lesions, DNA double-strand breaks (DSBs) are known as the most deleterious type of DNA damage due to the absence of an intact complementary strand for a template to repair DNA lesions [1] . These DSBs are usually repaired by two major pathways: homologous recombination (HR) and non-homologous end-joining (NHEJ). DDR requires a number of proteins, including MRN complex, ATM and ATR [2] . ATM is one of the key components in the DDR that functions as a phosphatidylinositol 3-kinase-like kinase. In human, ATM mutations result in genome instability syndromes, including cerebellar degeneration, immunodeficiency, radiation sensitivity and lymphoid tumours [3] . To repair DSBs, ATM should be activated by other proteins via direct (Tip60 acetyl-transferase and MRN [4] , [5] , [6] ) or indirect ways (Skp2 E3 ubiquitin ligase, 53BP1 and BRCA1 (refs 7 , 8 )). The activated ATM phosphorylates many downstream target proteins, one of which is Histone 2AX (H2Av in Drosophila ). Phosphorylated H2AX (γ-H2AX) enhances DNA repair efficiency by working as a platform to recruit various DNA repair proteins, histone modifiers and chromatin remodelers [1] , [9] . Drosophila ATM (dATM) has been extensively studied to understand its roles in genome stability and development. dATM mutants also show similar phenotypes associated with ATM patients such as neurodegeneration [10] , [11] , abnormal telomere protection [12] , [13] , increased apoptosis and chromosome fragmentation by DSB repair defects [10] , [11] , [13] , [14] , [15] . Additionally, dATM participates in silencing the expression of genes adjacent to telomere ends (telomere position effect) [16] , [17] and in alternative splicing of pre-messenger RNA [18] . In Drosophila, although genetic evidence suggests that dATM is positively regulated by MRN [19] and negatively by histone deacetylase ( RPD3 ) [10] , little is known how dATM is activated biochemically. Translationally controlled tumour protein (TCTP) is another highly conserved protein implicated in cancer and diverse cell functions ranging from cytoskeletal regulation to transcription [20] , [21] , [22] , [23] , [24] . Previously, we have shown that Drosophila TCTP (dTCTP) is essential for cell growth and proliferation by regulating TOR signalling [25] . Similar conserved roles for TCTP in growth regulation have also been found in plant and mammalian species [26] , [27] , [28] . In our search for new functions of dTCTP, we have found that dATM is a direct binding partner for dTCTP as described in this work. Interestingly, a recent study has suggested that human TCTP (hTCTP) plays a role for DNA damage control in fibroblast [29] . hTCTP is proposed as a target of ATM (ataxia telangiectasia-mutated) kinase because hTCTP is upregulated by IR and this upregulation is suppressed by ATM depletion. hTCTP forms a complex with ATM in an IR dose-dependent manner, and is known to be involved in the nuclear localization of Ku subunits of DNA-dependent protein kinase for NHEJ repair. However, several key questions on the nature of the interaction between ATM and hTCTP remained to be addressed. For example, it is not clearly defined whether hTCTP is required to regulate ATM kinase activity, stabilize binding between ATM and substrate or regulate subcellular distribution of ATM. One of the most important questions is whether hTCTP directly regulates ATM activity in response to DNA damages or interacts with other factors that function downstream to ATM. Since much of the work on hTCTP have been carried out in cell cultures, it is also important to investigate in vivo TCTP functions in genetic model organisms. Hence, comprehensive analysis of TCTP functions by genetic and biochemical approaches is necessary for understanding of the precise function of TCTP in the ATM pathway. In this study, we show that dTCTP plays important functions in the DDR and in cell cycle checkpoint control during organ development. Furthermore, we address key questions regarding the association between dTCTP and dATM. We show that dTCTP directly interacts with dATM and enhances the binding affinity of dATM to its substrate (H2Av), which facilitates dATM kinase activity and promotes efficient DNA repair. This is the first in vivo study to demonstrate direct regulation of ATM kinase activity by TCTP and its effect on genome stability. We thus provide new insights into the function of TCTP in normal development and cancer. Identification of dATM as a direct binding partner for dTCTP In order to find additional roles of dTCTP in Drosophila development, we have performed a phage display screen to identify new binding partners for dTCTP. In this screen of a random peptide library using an in vitro selection process [30] , we have found peptide heptamers containing the KCCYATK sequence that binds to dTCTP. Interestingly, one of the Drosophila proteins containing this peptide sequence was dATM. The carboxy-terminal PI3K-like kinase domain of ATM protein is highly conserved. On the contrary, the large amino-terminal region of ATM has only sparse sequence homology, and relatively little is known about the function of this region, except that it has a series of HEAT repeat domains [31] . The heptamer-matching region of dATM protein (1097–1101 amino-acid (aa) region) showed 71% sequence similarity (57% identity) with the heptamer according to the BLASTP algorithm ( Fig. 1a , the grey boxes under asterisk). This region seems to be a part of large helical structure consisting of multiple HEAT repeat domains acting as scaffolds for protein–protein interaction [31] . 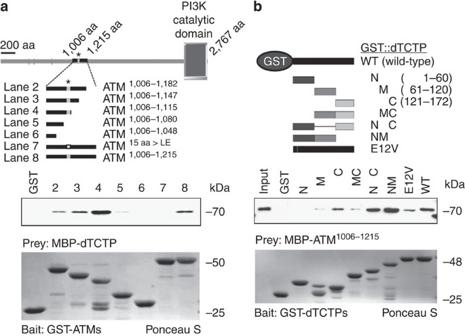Figure 1: Physical interactions between dTCTP and dATM. (a)In vitro, dTCTP directly binds to the dATM polypeptide fragment (black bar, 210 aa in length; Lane 8) and truncated dATM variants (Lanes 2–4) containing a short peptide sequence (FLCYSTK) with homology to dTCTP-interacting peptide heptamer (KCCYATK, grey boxes under asterisk). dTCTP shows considerably reduced binding to dATM fragments that are deleted in the heptamer binding region (Lanes 5–7). Lane 7 is a substitution variant in which a stretch of 15 aa covering the heptamer-matching region is replaced with LE (a white box). (b)In vitro, both M and C regions of dTCTP, but not an N region, are required for direct binding to the 210 aa region of dATM protein (Lanes N, M, C, and MC). The dTCTP N region seems to enhance the binding affinity between dTCTP and the dATM polypeptide (Lanes NC, NM and E12V). All experiments were performed in triplicate. Figure 1: Physical interactions between dTCTP and dATM. ( a ) In vitro , dTCTP directly binds to the dATM polypeptide fragment (black bar, 210 aa in length; Lane 8) and truncated dATM variants (Lanes 2–4) containing a short peptide sequence (FLCYSTK) with homology to dTCTP-interacting peptide heptamer (KCCYATK, grey boxes under asterisk). dTCTP shows considerably reduced binding to dATM fragments that are deleted in the heptamer binding region (Lanes 5–7). Lane 7 is a substitution variant in which a stretch of 15 aa covering the heptamer-matching region is replaced with LE (a white box). ( b ) In vitro , both M and C regions of dTCTP, but not an N region, are required for direct binding to the 210 aa region of dATM protein (Lanes N, M, C, and MC). The dTCTP N region seems to enhance the binding affinity between dTCTP and the dATM polypeptide (Lanes NC, NM and E12V). All experiments were performed in triplicate. Full size image To confirm that dTCTP physically interacts with dATM protein, we performed in vitro pull-down assay using a 210 aa region of dATM protein that includes the heptamer-matching region ( Fig. 1a ; the grey boxes under asterisk). MBP-dTCTP directly bound to this 210 aa region of dATM. Truncated ATM variants containing the heptamer-matching region showed the binding to dTCTP ( Fig. 1a ; Lanes 2–4 and 8). In contrast, mutated dATM proteins, in which the heptamer-matching region is deleted or substituted, showed much less binding to dTCTP ( Fig. 1a ; Lanes 5–7). Hence, these results suggest that the heptamer region is necessary for binding dTCTP. Additional tests with truncated dTCTP proteins indicated that the direct binding between dTCTP and a 210 aa region of dATM is mediated by the middle and C-terminal parts of dTCTP ( Fig. 1b ; Lanes M, C and MC) but not by N-terminal region ( Fig. 1b ; Lane N). Interestingly, although the N-terminal region does not bind to dATM, its presence appears to promote the binding between dTCTP and dATM by an unknown mechanism (Lanes M, C, MC versus NC, NM, WT). In addition, the E12 substitution (E12 to V) in the N-terminal region of dTCTP, which critically impairs the dTCTP function [25] , considerably reduced the level of binding to dATM (dTCTP E12V Lane). Structurally, TCTP is divided into three regions: β-strands in N-terminus, helices in the middle and flexible loop in C-terminus [20] . Thus, these results suggest that the helical and flexible loop regions of dTCTP is required to form a protein complex with dATM in vitro by specific and direct binding. Nuclear chromatin localization of dTCTP protein Previously, we reported that dTCTP regulates cell growth in Drosophila imaginal discs by regulating TOR signalling [25] . Thus, in parallel with the peptide screen, we have also examined the role of dTCTP for growth regulation in salivary glands, a well-known model organ for studying cell growth [32] . In this study, we unexpectedly found that considerable levels of dTCTP protein are located in the cell nucleus of the salivary glands and fat bodies ( Fig. 2a,b , arrowheads). Western blot analysis on cytosolic and nuclear fractions from embryo extract also confirmed this nuclear localization of dTCTP protein ( Fig. 2c ). Furthermore, dTCTP protein in the salivary gland cell nucleus was found to be associated with polytene chromosomes in the wild-type. In contrast, dTCTP staining was greatly reduced or absent in polytene chromosomes from dTCTP EY09182 hypomorphic mutant, indicating the specificity of this chromosomal localization ( Fig. 2d ). 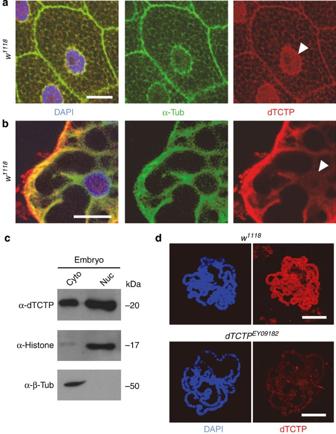Figure 2: Nuclear localization of dTCTP. (a,b) dTCTP proteins (red) are localized in cell nuclei (arrowheads) of both salivary gland (a) and fat body (b) from wild-type (w1118) larva. dTCTP is also overlapped with α-tubulin (green). Cell nuclei are stained with DAPI (blue). Scale bar, 20 μm. (c) dTCTP western blot on cytosolic and nuclear fractions of wild-type embryo extract. Histone and β-tubulin antibodies were used as quality controls of nuclear and cytosolic fractions, respectively. (d) Chromosomes stained with DAPI and anti-dTCTP antibody. (upper panels) dTCTP is localized to polytene chromosomes from salivary gland cells of third instar wild-type larvae. (lower panels) dTCTP staining in homozygousdTCTPEY09182(strong hypomorph) polytene chromosomes is greatly reduced. All experiments were performed in triplicate. Scale bar, 40 μm. Figure 2: Nuclear localization of dTCTP. ( a , b ) dTCTP proteins (red) are localized in cell nuclei (arrowheads) of both salivary gland ( a ) and fat body ( b ) from wild-type ( w 1118 ) larva. dTCTP is also overlapped with α-tubulin (green). Cell nuclei are stained with DAPI (blue). Scale bar, 20 μm. ( c ) dTCTP western blot on cytosolic and nuclear fractions of wild-type embryo extract. Histone and β-tubulin antibodies were used as quality controls of nuclear and cytosolic fractions, respectively. ( d ) Chromosomes stained with DAPI and anti-dTCTP antibody. (upper panels) dTCTP is localized to polytene chromosomes from salivary gland cells of third instar wild-type larvae. (lower panels) dTCTP staining in homozygous dTCTP EY09182 (strong hypomorph) polytene chromosomes is greatly reduced. All experiments were performed in triplicate. Scale bar, 40 μm. Full size image dTCTP forms a protein complex and nuclear foci with dATM The findings that dTCTP binds to a fragment of nuclear protein dATM and is expressed in endocycling cells such as salivary glands and fat cells prompted us to test in vivo interaction between dTCTP and dATM. First, we performed co-immunoprecipitation (co-IP) using S2 cells transfected with FLAG-dATM and MYC-dTCTP. We also expressed V5-tagged Drosophila Rad50 and Mre11, because Mre11 and Rad50 (MR complex) are known to form a functional complex with ATM in mammals [5] , [6] . In both reciprocal co-IP using MYC antibody (for dTCTP) and FLAG antibody (for dATM), dTCTP was found to be associated with dATM and MR complex ( Fig. 3a ; Lanes 4–6). Furthermore, dTCTP was also co-immunoprecipitated with dATM in wild-type pupal nuclear extracts (NEs), while such interaction was substantially reduced in dTCTP EY / h59 mutants ( Fig. 3b , upper panels). The interaction between dTCTP and dATM was resistant to the treatment with benzonase ( Supplementary Fig. S1 ). These results indicate that dTCTP forms a specific protein complex with dATM in vivo . 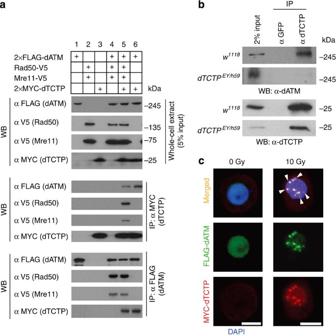Figure 3: dTCTP forms a protein complex and nuclear foci with dATM. (a) In S2 cell, dTCTP is co-immunoprecipitated with both dATM and dATM-MR complex (Lanes 5, 6). Reciprocal co-IPs were performed using anti-MYC (middle panels) or anti-FLAG (bottom panels). (b)In vivo, dTCTP is co-immunoprecipitated with dATM in NE from wild-type pupae, but much less in extract fromdTCTPEY/h59mutants (upper panels). (c) γ-irradiation induces the formation of dATM foci. A subset of dTCTP foci can co-localize with that of dATM (white arrowheads). S2 cells were transiently transfected with expression vectors containing FLAG-dATM and MYC-dTCTP. All experiments were performed in triplicate. Scale bars, 5 μm. Figure 3: dTCTP forms a protein complex and nuclear foci with dATM. ( a ) In S2 cell, dTCTP is co-immunoprecipitated with both dATM and dATM-MR complex (Lanes 5, 6). Reciprocal co-IPs were performed using anti-MYC (middle panels) or anti-FLAG (bottom panels). ( b ) In vivo , dTCTP is co-immunoprecipitated with dATM in NE from wild-type pupae, but much less in extract from dTCTP EY/h59 mutants (upper panels). ( c ) γ-irradiation induces the formation of dATM foci. A subset of dTCTP foci can co-localize with that of dATM (white arrowheads). S2 cells were transiently transfected with expression vectors containing FLAG-dATM and MYC-dTCTP. All experiments were performed in triplicate. Scale bars, 5 μm. Full size image To further confirm these interactions, we checked nuclear colocalization and foci formation between dATM and dTCTP in S2 cell following γ-irradiation. Overexpressed FLAG-dATM in S2 cell was preferentially localized to the cell nucleus with few foci, whereas the level of nuclear MYC-dTCTP was very low ( Fig. 3c , 0 Gy). However, after 10 Gy of γ-irradiation on the S2 cells, both proteins were colocalized in the cell nucleus and formed nuclear foci ( Fig. 3c ). Interestingly, when dATM level was depleted in S2 cell using atm RNA interference (RNAi) ( Supplementary Fig. S2A ), dTCTP foci formation following γ-irradiation was dramatically diminished, although dTCTP can still translocate into cell nucleus ( Supplementary Fig. S2E ). However, in the case of dTCTP depletion ( Supplementary Fig. S2B ), dATM foci were properly formed responding to γ-irradiation ( Supplementary Fig. S2D ). This result suggests that dATM is required for dTCTP to form IR-induced foci but not vice versa . Altogether, these results show that both dTCTP and dATM can form a protein complex in vivo , and they may cooperate on DSB repair processes at the sites of nuclear foci induced by γ-irradiation. Radiation sensitivity in dTCTP mutants Our biochemical and histochemical data suggest that dTCTP may be involved in the control of genome stability by forming a protein complex with dATM through direct interaction. If dTCTP is required for genome stability, we expect that dTCTP mutants would show higher radiation sensitivity upon γ-irradiation compared with wild-type. To attest this idea, we examined adult viability, morphology change and chromosome instability in dTCTP mutants following γ-irradiation. To study the effects of radiation on the survival of third instar larvae and adult mutants, we used a hypomorphic condition in dTCTP EY09182 / dTCTP h59 ( dTCTP EY / h59 in short) transheterozygotes since dTCTP h59 -null mutants die too early to measure the radiation effects. dTCTP EY / h59 flies show substantially reduced protein level ( Fig. 4a ), indicating that this allelic combination represents a strong hypomorphic condition. As expected, γ-irradiated dTCTP EY / h59 -mutant adults showed considerably higher dose-dependent radiation sensitivity than wild-type flies, and this high sensitivity in dTCTP mutants was fully restored by introducing the TCTP Ge30-2 genomic transgene ( Fig. 4b–d ). 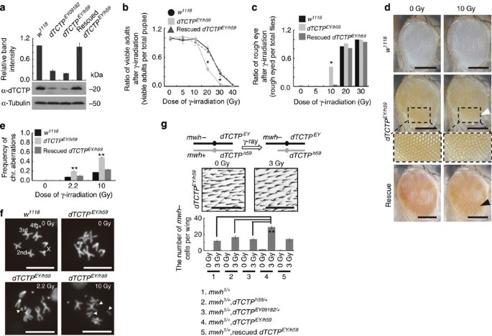Figure 4: Ionizing radiation (IR) sensitivity indTCTPmutants. (a)dTCTPtransheterozygote mutant,dTCTPEY09182/dTCTPh59(dTCTPEY/h59) is a strong hypomorph. dTCTP western blot band intensity is normalized to α-tubulin. dTCTP expression levels in homozygousdTCTPEY09182anddTCTPEY/h59adult flies are reduced to 27 and 20% of wild-type level, respectively. dTCTP expression indTCTPEY/h59mutant is restored by introducing a genomic fragment ofdTCTP (dTCTPGe30-2). Performed in triplicate. Error bars indicate s.e.m. (b) Reduced viability ofdTCTPEY/h59mutants following different doses of γ-irradiation. The IR sensitivity ofdTCTPEY/h59mutants is rescued bydTCTPGe30-2. Performed in octaplicate. Error bars indicate s.e.m. *P<0.005 (t-test). (c,d) Rough eye phenotypes following different doses of γ-irradiation. High doses of IR (20 and 30 Gy) cause rough eye phenotypes in all genotypes (wild-type,dTCTPEY/h59and rescueddTCTPmutants bydTCTPGe30-2), while at 10 Gy, onlydTCTPEY/h59mutants show rough eyes (c, *P<0.005 (t-test) andd, white arrowhead). Note that ommatidial arrays are irregular indTCTPEY/h59mutants (rectangles with dotted line).n⩾200. Scale bars, 200 μm. (e–g) DSB repair defects increase indTCTPmutants by γ-irradiation. (e) Metaphase chromosome spreads from neuroblasts in larval brain. Chromosome aberrations are more frequent after γ-irradiation indTCTPEY/h59mutants, compared with wild-type ( 2.8-fold at 2.2 Gy and 2.4-fold at 10 Gy); **P<0.0001 (t-test). (f) Representatives of panel E. Broken chromosomal arms are seen indTCTPEY/h59mutant (arrowheads). Performed in triplicate. Scale bars, 10 μm. (g) Increased loss of heterozygosity detected by themwh-mutant phenotype after γ-irradiation ofdTCTP-mutant larvae. After IR treatment (3 Gy), chromosome breaks indicated indirectly by themwh-mutant phenotype are increased indTCTPmutants (asterisk, #4) compared with both wild-type (#1) anddTCTPheterozygotes (#2 and 3) (about 2.4 and 1.8 or 2.0-folds, respectively).dTCTP-mutant phenotype is rescued bydTCTPGe30-2(#5). Over 10 adult wings were measured for each experiment. Performed in triplicate. **P<0.0001 (t-test). All error bars indicate s.e.m. Scale bars, 50 μm. Figure 4: Ionizing radiation (IR) sensitivity in dTCTP mutants. ( a ) dTCTP transheterozygote mutant, dTCTP EY09182 /dTCTP h59 ( dTCTP EY/h59 ) is a strong hypomorph. dTCTP western blot band intensity is normalized to α-tubulin. dTCTP expression levels in homozygous dTCTP EY09182 and dTCTP EY/h59 adult flies are reduced to 27 and 20% of wild-type level, respectively. dTCTP expression in dTCTP EY/h59 mutant is restored by introducing a genomic fragment of dTCTP (dTCTP Ge30-2 ). Performed in triplicate. Error bars indicate s.e.m. ( b ) Reduced viability of dTCTP EY/h59 mutants following different doses of γ-irradiation. The IR sensitivity of dTCTP EY/h59 mutants is rescued by dTCTP Ge30-2 . Performed in octaplicate. Error bars indicate s.e.m. * P <0.005 ( t -test). ( c , d ) Rough eye phenotypes following different doses of γ-irradiation. High doses of IR (20 and 30 Gy) cause rough eye phenotypes in all genotypes (wild-type, dTCTP EY/h59 and rescued dTCTP mutants by dTCTP Ge30 -2 ), while at 10 Gy, only dTCTP EY/h59 mutants show rough eyes ( c , * P <0.005 ( t -test) and d , white arrowhead). Note that ommatidial arrays are irregular in dTCTP EY/h59 mutants (rectangles with dotted line). n ⩾ 200. Scale bars, 200 μm. ( e – g ) DSB repair defects increase in dTCTP mutants by γ-irradiation. ( e ) Metaphase chromosome spreads from neuroblasts in larval brain. Chromosome aberrations are more frequent after γ-irradiation in dTCTP EY/h59 mutants, compared with wild-type ( 2.8-fold at 2.2 Gy and 2.4-fold at 10 Gy); ** P <0.0001 ( t -test). ( f ) Representatives of panel E. Broken chromosomal arms are seen in dTCTP EY/h59 mutant (arrowheads). Performed in triplicate. Scale bars, 10 μm. ( g ) Increased loss of heterozygosity detected by the mwh -mutant phenotype after γ-irradiation of dTCTP- mutant larvae. After IR treatment (3 Gy), chromosome breaks indicated indirectly by the mwh -mutant phenotype are increased in dTCTP mutants (asterisk, #4) compared with both wild-type (#1) and dTCTP heterozygotes (#2 and 3) (about 2.4 and 1.8 or 2.0-folds, respectively). dTCTP- mutant phenotype is rescued by dTCTP Ge30-2 (#5). Over 10 adult wings were measured for each experiment. Performed in triplicate. ** P <0.0001 ( t -test). All error bars indicate s.e.m. Scale bars, 50 μm. Full size image One of the major effects of IR is DSBs in the chromatin [2] . Thus, we inferred that the higher IR sensitivity in dTCTP mutants may be due to increased incidents of DSB in their chromatin. We tested this possibility by utilizing two sensitive assays for indirectly detecting DSB repair defects resulting from low levels of irradiation [2] , [33] , [34] . One is to examine chromosomal aberrations in larval brain neuroblasts, and the other is to measure the level of chromosome breaks in adult wings based on the loss of heterozygosity for a distal genetic marker multiple wing hair (mwh) following γ-irradiation. Indeed, mitotic chromosomes from both larval brain neuroblasts and adult wing hair cells revealed more than twofold higher levels of DSB repair defects in dTCTP mutants than the wild-type or heterozygous controls ( Fig. 4e–g , asterisks or arrowheads). On the contrary, spontaneous chromosome aberrations in the absence of γ-irradiation were absent in wild-type and very low in dTCTP mutants ( Supplementary Table S1 ). These IR-sensitive phenotypes in dTCTP mutants were rescued by introducing a copy of dTCTP Ge30-2 genomic fragment. In addition to the enhanced IR-induced genome instability, abnormal patterns of mitosis were detected in early dTCTP mutant embryos derived from homozygous dTCTP EY09182 females that have little maternal dTCTP. These mutant embryos showed various mitotic defects such as chromosomal bridges and free centrosomes due to the falling of nuclei from the periphery of the embryo ( Supplementary Fig. S3 ) [14] , [15] , [35] , [36] . Thus, these high sensitivities to induced and uninduced DSBs in dTCTP mutants strongly suggest that, at the whole-organism level, dTCTP is required to maintain genome stability in various tissue types and developmental stages, especially through DSB repair process that depends on ATM protein. Replication and G2/M checkpoints defects in dTCTP mutants DNA damage triggers checkpoint responses such as cell cycle arrest to repair DNA damage or apoptosis to remove irreversibly damaged cells [37] . In dTCTP mutants, induced DSBs result in genome instability, or increased radiation sensitivity ( Fig. 4 ). Thus, we examined whether induced DSBs in dTCTP mutants cause improper checkpoint responses. dTCTP mutants were examined by labelling of developing organs with phospho-histone H3 (PH3), BrdU and terminal deoxynucleotidyl transferase dUTP nick end labeling (TUNEL) to evaluate G2/M, intra S checkpoints and apoptosis, respectively. These assays revealed that cell cycle arrests are impaired in somatic and neuronal cells of dTCTP mutants ( Fig. 5a,b and Supplementary Fig. S4 ). These impairments result in more apoptosis in dTCTP mutants to remove damaged cell ( Fig. 5c ). 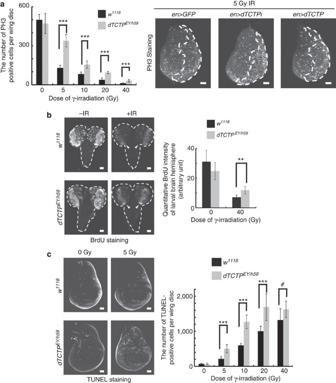Figure 5: DNA damage responses indTCTPmutants. (a) G2/M checkpoint defect indTCTPEY/h59mutants after γ-irradiation. Third instar larvae treated by IR were rested for 1 h, and mitotic cells in wing discs were visualized with phospho-histone 3 antibody (PH3). (Left Histogram) after γ-irradiation, the numbers of mitotic cells indTCTPmutants are higher compared with wild-type.n=13. ***P<0.0001 (t-test). Error bars are s.d. (Right panels)dTCTPRNAi (dTCTPi) or dTCTP overexpression in the posterior compartment of wing disc usingen-GAL4driver. Five Gy of IR leads to reduced PH3 puncta in both anterior and posterior compartments ofen>GFPanden>dTCTP, while the posterior compartment ofen>dTCTPishows much less reduction of PH3 puncta.n=12. All experiments were performed in duplicate. Scale bars, 50 μm. (b) Intra S checkpoint defect indTCTPEY/h59mutant, reared for 1.5 h after IR. RDS is seen in larval brain hemispheres ofdTCTPmutants (arrowheads). Intra S checkpoint arrest is significantly less indTCTPmutant. Error bars are s.d.n=11. **P<0.001 (t-test). Performed in duplicate. Scale bars, 50 μm. (c) Apoptosis (TUNEL assay) in wing disc cells from wild-type anddTCTPEY/h59, reared for 4 h after γ-irradiation.dTCTPmutants show higher levels of apoptotic cells, compared with wild-type. Error bars are s.d.n=10. ***P<0.0001.#P>0.05 (t-test). Performed in duplicate. Scale bars, 50 μm. Figure 5: DNA damage responses in dTCTP mutants. ( a ) G2/M checkpoint defect in dTCTP EY/h59 mutants after γ-irradiation. Third instar larvae treated by IR were rested for 1 h, and mitotic cells in wing discs were visualized with phospho-histone 3 antibody (PH3). (Left Histogram) after γ-irradiation, the numbers of mitotic cells in dTCTP mutants are higher compared with wild-type. n =13. *** P <0.0001 ( t -test). Error bars are s.d. (Right panels) dTCTP RNAi ( dTCTPi ) or dTCTP overexpression in the posterior compartment of wing disc using en-GAL4 driver. Five Gy of IR leads to reduced PH3 puncta in both anterior and posterior compartments of en>GFP and en > dTCTP , while the posterior compartment of en>dTCTPi shows much less reduction of PH3 puncta. n =12. All experiments were performed in duplicate. Scale bars, 50 μm. ( b ) Intra S checkpoint defect in dTCTP EY/h59 mutant, reared for 1.5 h after IR. RDS is seen in larval brain hemispheres of dTCTP mutants (arrowheads). Intra S checkpoint arrest is significantly less in dTCTP mutant. Error bars are s.d. n =11. ** P <0.001 ( t -test). Performed in duplicate. Scale bars, 50 μm. ( c ) Apoptosis (TUNEL assay) in wing disc cells from wild-type and dTCTP EY/h59 , reared for 4 h after γ-irradiation. dTCTP mutants show higher levels of apoptotic cells, compared with wild-type. Error bars are s.d. n =10. *** P <0.0001. # P >0.05 ( t -test). Performed in duplicate. Scale bars, 50 μm. Full size image G2/M arrest was prominent in wild-type wing discs after IR, while such arrest was much reduced in dTCTP mutant, resulting in about 2–2.5-fold greater mitotic cells than wild-type ( Fig. 5a , histogram). Especially, at a low dose of IR (5 Gy), this difference between wild-type and the mutant was more pronounced (2.6-fold). To further confirm this, we knocked down dTCTP expression only in the posterior compartment of wing disc using engrailed-Gal4 ( en>dTCTPi, dTCTP RNAi), and the anterior compartment of the wing disc was used as an internal control ( Fig. 5a , right panels). At 5 Gy of IR, cell cycle arrest in wing discs from en>GFP control reduced mitotic cell numbers in both compartments. In contrast, the number of mitotic cells from en>dTCTPi did not significantly decrease in the posterior compartment, indicating that G2/M arrest after IR is compromised only in the posterior by dTCTP knockdown. We also found that irradiated dTCTP mutants showed impaired S-phase checkpoint when radioresistant DNA synthesis (RDS) response was assayed by BrdU incorporation in larval brain ( Fig. 5b , arrowheads and Supplementary Fig. S4 ). Improper cell cycle arrest results in apoptosis to remove cells with permanently damaged genomic DNA [37] . As expected from radiation sensitivity and impaired cell cycle arrest in dTCTP mutants, induced DSBs in dTCTP EY / h59 mutants caused about twofold greater cell death at 5, 10 and 20 Gy of IR compared with the wild-type control levels ( Fig. 5c , 2.4, 2.1 and 1.7-folds, respectively). At 40 Gy, the number of dead cells was not significantly different ( P >0.05, t -test), although higher than that of wild-type. Taken together, these data suggest that dTCTP mutants improperly respond to induced DSBs at the cellular level, and that dTCTP mutations probably affect the early steps of DDR such as DSB signal propagation, since dTCTP makes a protein complex with dATM and atm mutants partially share similar responses with dTCTP mutants [14] , [15] , [38] . dTCTP genetically interacts with dATM and other DDR genes The direct interaction between dTCTP and dATM ( Figs 1 and 3 ) and the roles of dTCTP in genome stability at the whole organism and cellular levels ( Figs 4 and 5 ) led us to ask whether dTCTP is functionally associated with dATM in vivo using genetic approaches. Indeed, we found strong genetic interactions in transheterozygotes or hypomorphic conditions for dTCTP and atm mutations. First, the pupation start time is considerably delayed by 2 days. Wild-type, +/atm (strong hypomorphic atm 3 or null atm 6 alleles; Supplementary Fig. S5C,D ) or +/dTCTP (strong hypomorphic dTCTP EY09182 and null dTCTP h59 alleles) heterozygote controls showed 100% eclosion at 5 days after puparium formation. However, it took 7 days for transheterozygotes for both dTCTP and atm mutations ( Fig. 6a , blue and orange bars). 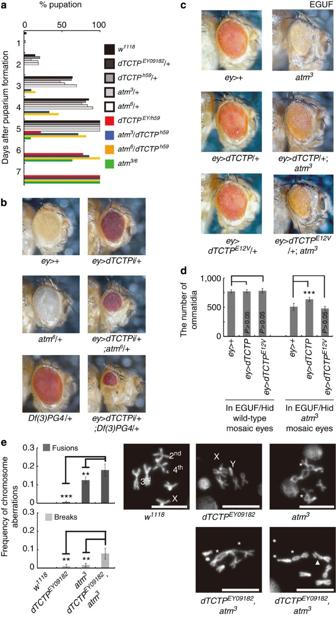Figure 6: Genetic interaction betweendTCTPandatm. (a) The pupation start time in the transheterozygotes ofdTCTPandatm(atm3/dTCTPh59andatm6/dTCTPh59) is delayed for ~2 days, compared with wild-type or heterozygotes for eitherdTCTPoratm.atm3/6mutants show pupal lethality. Eggs deposited for 2 days by mated young females were developed in cornmeal media.n=100–120. Performed in triplicate.atm3anddTCTPEY09182are strong hypomorphic alleles.atm6anddTCTPh59are null alleles. (b) Heterozygotes foratm6(right middle panel) oratmdeficiencyDf(3)PG4(right lower panel) enhance the small eye phenotype ofey>dTCTPiflies. (c) Small eye phenotypes of EGUF/Hid strong hypomorphicatm3mosaic eyes are partially rescued by increasing dTCTP expression (right middle panel). Overexpression of a point-mutateddTCTPtransgene,UAS-dTCTPE12V, shows no rescue effect compared withdTCTPoverexpression (right lower panel). (d) Quantitative analysis of panelc. Error bars indicate s.d. ***P<0.0001 (t-test). The number of ommatidia was scored from 10 adult eyes for each genotype. (e) Rates of spontaneous DSBs are notably increased in the larval neuroblasts ofdTCTPEY09182, atm3double hypomorphic-mutant homozygote, compared with the single mutant homozygote of each gene. Representative phenotypes for each genotype are shown. Asterisk: fused chromosome arm. Arrowhead: Chromosome break. Performed in triplicate. Over 300 neuroblasts were examined. ***P<0.001 and **P<0.01 (t-test). Error bars indicate s.d. Scale bars, 10 μm. Figure 6: Genetic interaction between dTCTP and atm. ( a ) The pupation start time in the transheterozygotes of dTCTP and atm ( atm 3 /dTCTP h59 and atm 6 /dTCTP h59 ) is delayed for ~2 days, compared with wild-type or heterozygotes for either dTCTP or atm . atm 3/6 mutants show pupal lethality. Eggs deposited for 2 days by mated young females were developed in cornmeal media. n =100–120. Performed in triplicate. atm 3 and dTCTP EY09182 are strong hypomorphic alleles. atm 6 and dTCTP h59 are null alleles. ( b ) Heterozygotes for atm 6 (right middle panel) or atm deficiency Df(3)PG4 (right lower panel) enhance the small eye phenotype of ey>dTCTPi flies. ( c ) Small eye phenotypes of EGUF/Hid strong hypomorphic atm 3 mosaic eyes are partially rescued by increasing dTCTP expression (right middle panel). Overexpression of a point-mutated dTCTP transgene, UAS-dTCTP E12V , shows no rescue effect compared with dTCTP overexpression (right lower panel). ( d ) Quantitative analysis of panel c . Error bars indicate s.d. *** P <0.0001 ( t -test). The number of ommatidia was scored from 10 adult eyes for each genotype. ( e ) Rates of spontaneous DSBs are notably increased in the larval neuroblasts of dTCTP EY09182 , atm 3 double hypomorphic-mutant homozygote, compared with the single mutant homozygote of each gene. Representative phenotypes for each genotype are shown. Asterisk: fused chromosome arm. Arrowhead: Chromosome break. Performed in triplicate. Over 300 neuroblasts were examined. *** P <0.001 and ** P <0.01 ( t -test). Error bars indicate s.d. Scale bars, 10 μm. Full size image We also found strong genetic interaction between dTCTP and atm in eye development. First, one copy deletion of atm gene (+/Df(3)PG4 ) or atm heterozygotes (+/atm 6 ) dramatically enhanced the small eye phenotype caused by expressing dTCTP RNAi ( ey > dTCTPi ) ( Supplementary Table S2 and Fig. 6b ). Next, we increased the amount of dTCTP in atm 3 hypomorphic or atm 6 null mutant eyes to further confirm the genetic interaction between the two genes. EGUF/Hid technique [39] was used to remove most wild-type cells by eye-specific cell death in atm mosaic eyes, and then dTCTP was expressed using ey-GAL4 in EGUF/Hid atm mosaic eyes. Similar to a previous report [14] , EGUF/Hid atm mosaic eyes showed a reduced eye size ( Fig. 6c , right upper panel and d; Supplementary Fig. S5A,B ). Interestingly, dTCTP overexpression in atm 3 mosaic eyes strongly suppressed their reduced eye phenotypes ( Fig. 6c , right middle panel and d), while overexpression of a mutated dTCTP (dTCTP E12V ) did not ( Fig. 6c , right lower panel and d). This result indicates that dTCTP can promote the function of dATM and supports the importance of this E12 residue for the TCTP interaction with ATM ( Fig. 1b ). Notably, in contrast to hypomorphic atm 3 mosaic eye, the null atm 6 mosaic eye phenotype was not suppressed by overexpressing dTCTP ( Supplementary Fig. S5A,B ), suggesting that dTCTP is unable to promote dATM activity in the dATM-null condition. Consistent with genetic interactions in the eye, we observed functional association between dTCTP and atm ( Fig. 6e ). Chromosome aberrations in neuroblasts of larval brain were examined in two single hypomorphic-mutant homozygotes ( dTCTP EY09182 or atm 3 ) and in a double hypomorphic homozygote ( dTCTP EY09182 , atm 3 ). Similar to previous reports [12] , [14] , [15] , homozygous atm 3 mutants showed chronic spontaneous chromosome aberrations ( Fig. 6e ; 12.5% of fused chromosomal arms and 1.6% of DSBs), while dTCTP EY09182 hypomorphic homozygotes showed much lower levels of chromosome aberrations (0.6 and 1.0%). Intriguingly, double hypomorphic-mutant homozygote ( dTCTP EY09182 , atm 3 ) showed increased chromosome aberrations (18.0 and 7.9%), in which DSBs were remarkably increased (4.9-fold) compared with atm 3 homozygote. These results suggest that dTCTP plays a role in the DSB repair process by interacting with dATM. To further support the function of dTCTP in DSB repair, we mated ey > dTCTPi flies with RNAi lines or mutant alleles for DDR genes and examined their effects on the eye size to test whether dTCTP interacts with other DDR genes. The MRN complex (Mre11-Rad50-Nbs1) is a DSB sensor and is important for both HR and NHEJ [9] . When each component of MRN complex was reduced by RNAi expression or a recessive mutant allele in the ey>dTCTPi background, the eye sizes of ey > dTCTPi flies were significantly reduced ( Supplementary Fig. S6A , Supplementary Table S2 ). Likewise, dTCTP genetically interacted with other HR-associated genes ( His2Av , MDC1 and MCPH1 ) as well as NHEJ-associated genes ( Lig4 and ku70 ) ( Supplementary Fig. S6B,C , Supplementary Table S2 ). However, dTCTP showed little genetic interactions with the genes involved in base excision or DNA single-strand breaks repair process ( Supplementary Table S2 ). Taken together, these data suggest that dTCTP is specifically required for DSB repair in a dATM-dependent manner but not for SSB repair. dTCTP is required for efficient H2Av phosphorylation Upon DNA damages, mammalian and Drosophila ATMs are recruited to the damaged sites to form nuclear foci at the DSB sites [1] , [9] , [11] ( Supplementary Fig. S8 ). At the foci, ATM phosphorylates histone 2A variants (γ-H2AX in mammals and γ-H2Av in flies) to facilitate DSB repair processes. Our data for physical and genetic interactions between dTCTP and dATM indicate that they cooperate positively for DSB repair. For example, dTCTP may act as a positive modulator for dATM enzyme activity. If this hypothesis is correct, we could expect to see a decreased level of γ-H2Av in the dTCTP mutants compared with wild-type. Thus, we checked whether dATM activity is impaired in dTCTP mutants by assaying γ-H2Av level of endocycling larval salivary gland cells. In wild-type, these cells have a large number of DSBs in their nuclei due to repeated replication [32] , resulting in high levels of H2Av phosphorylation. Immunohistochemistry and western blot analysis showed that γ-H2Av levels in homozygous dTCTP EY09182 ( dTCTP EY/EY ) and dTCTP EY/h59 mutants are considerably reduced to about half of the wild-type level ( Fig. 7a ). The reduced level of γ-H2Av in dTCTP EY/EY mutants was nearly comparable to that in the atm 3 strong hypomorph. ( Fig. 7b ). Therefore, these data suggest that dATM activity to phosphorylate H2Av responding to DSBs might be significantly affected by reducing dTCTP. 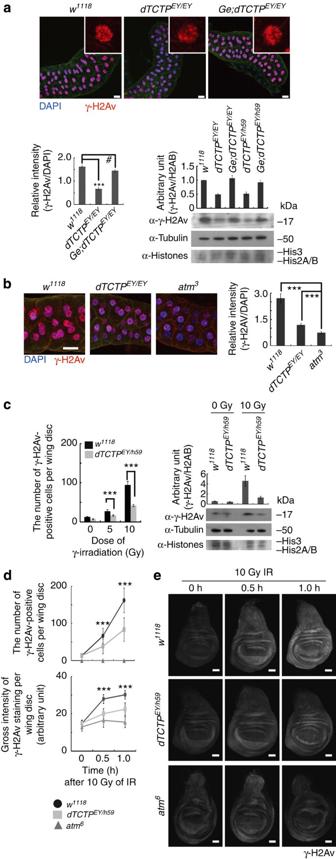Figure 7: dTCTP affects ATM kinase activityin vivo. (a) Reduction of nuclear γ-H2Av level (red) in third instar larval salivary gland ofdTCTPmutants. (Upper left) endocycling salivary gland cells have many DSBs in their nuclei (insets, γ-H2Av stained cell nuclei in a higher magnification). (Upper middle) reduced γ-H2Av level in homozygousdTCTPEY09182mutant (dTCTPEY/EY). (Upper right)dTCTPEY/EYmutants are rescued by the genomicdTCTPGetransgene (Ge;dTCTPEY09182). (Lower left) quantitative analysis of γ-H2Av intensity. γ-H2Av intensity was normalized by that of nuclear DAPI (blue). Salivary glands were counterstained by α-tubulin (green).n=20. Error bars are s.d. ***P<0.001.#P>0.02 (t-test). (Lower right) western blot analysis to detect γ-H2Av levels in wild-type and indicated genotypes. Relative band intensities were quantified (bar graphs). Error bars are s.e.m. Performed in triplicate. Scale bar, 40 μm. (b) Reduced γ-H2Av levels in salivary gland cells from bothdTCTPEY/EYandatm3mutants. Histogram indicates quantitative analysis of γ-H2Av intensity. Error bars are s.e.m. ***P<0.001 (t-test). Performed in triplicate. Scale bar, 40 μm. (c) (Left) γ-H2Av foci formation in IR-exposed wing discs. At 5 and 10 Gy of IR,dTCTPEY/h59mutants (grey bars) show low levels of γ-H2Av compared withw1118control (black bars). Third instar larvae treated with different doses of IR were rested for 1 h and dissected.n=9–12. Error bars are s.d. ***P<0.001 (t-test). (Right) western blot analysis in IR-exposed wing discs. Relative band intensities were quantified (bar graphs). Error bars are s.e.m. Performed in triplicate. (d,e) The kinetics of γ-H2Av foci formation and gross intensity change in IR-exposed wing discs fromw1118control,dTCTPEY/h59and homozygousatm6mutants. Third instar larvae treated with 10 Gy of IR were dissected at 0, 0.5 and 1 h after irradiation. γ-H2Av levels (both foci number and gross intensity) after irradiation inw1118control are significantly increased in a time-dependent manner (d). On the contrary, responding to irradiation,dTCTPEY/h59mutants show low increase in γ-H2Av levels. Homozygousatm6mutants show no significant changes in γ-H2Av levels.n=20. Error bars are s.d. ***P<0.001 (t-test) (e) Representatives of paneld. Scale bars, 50 μm. Figure 7: dTCTP affects ATM kinase activity in vivo . ( a ) Reduction of nuclear γ-H2Av level (red) in third instar larval salivary gland of dTCTP mutants. (Upper left) endocycling salivary gland cells have many DSBs in their nuclei (insets, γ-H2Av stained cell nuclei in a higher magnification). (Upper middle) reduced γ-H2Av level in homozygous dTCTP EY09182 mutant ( dTCTP EY / EY ). (Upper right) dTCTP EY/EY mutants are rescued by the genomic dTCTP Ge transgene ( Ge ; dTCTP EY09182 ). (Lower left) quantitative analysis of γ-H2Av intensity. γ-H2Av intensity was normalized by that of nuclear DAPI (blue). Salivary glands were counterstained by α-tubulin (green). n =20. Error bars are s.d. *** P <0.001. # P >0.02 ( t -test). (Lower right) western blot analysis to detect γ-H2Av levels in wild-type and indicated genotypes. Relative band intensities were quantified (bar graphs). Error bars are s.e.m. Performed in triplicate. Scale bar, 40 μm. ( b ) Reduced γ-H2Av levels in salivary gland cells from both dTCTP EY/EY and atm 3 mutants. Histogram indicates quantitative analysis of γ-H2Av intensity. Error bars are s.e.m. *** P <0.001 ( t -test). Performed in triplicate. Scale bar, 40 μm. ( c ) (Left) γ-H2Av foci formation in IR-exposed wing discs. At 5 and 10 Gy of IR, dTCTP EY/h59 mutants (grey bars) show low levels of γ-H2Av compared with w 1118 control (black bars). Third instar larvae treated with different doses of IR were rested for 1 h and dissected. n =9–12. Error bars are s.d. *** P <0.001 ( t -test). (Right) western blot analysis in IR-exposed wing discs. Relative band intensities were quantified (bar graphs). Error bars are s.e.m. Performed in triplicate. ( d , e ) The kinetics of γ-H2Av foci formation and gross intensity change in IR-exposed wing discs from w 1118 control, dTCTP EY/h59 and homozygous atm 6 mutants. Third instar larvae treated with 10 Gy of IR were dissected at 0, 0.5 and 1 h after irradiation. γ-H2Av levels (both foci number and gross intensity) after irradiation in w 1118 control are significantly increased in a time-dependent manner ( d ). On the contrary, responding to irradiation, dTCTP EY/h59 mutants show low increase in γ-H2Av levels. Homozygous atm 6 mutants show no significant changes in γ-H2Av levels. n =20. Error bars are s.d. *** P <0.001 ( t -test) ( e ) Representatives of panel d . Scale bars, 50 μm. Full size image The reduction of γ-H2Av level in salivary glands of dTCTP mutants could result from reduced endocycling by dTCTP defects. To circumvent this possibility, we tested whether γ-H2Av level is also reduced in the irradiated mitotic cells of dTCTP mutants. Consistent with the results from endocycling salivary cells, mitotic cells from both dTCTP mutants and dTCTP-depleted S2 cells also showed reduced H2Av phosphorylation activity responding to induced DSBs ( Fig. 7c–e and Supplementary Fig. S7 ). Imaginal discs from irradiated dTCTP EY/h59 mutants showed substantially less γ-H2Av-positive cells than wild-type (about 40 and 55% reduction at 5 Gy and 10 Gy, respectively). Similarly, the level of γ-H2Av was considerably diminished in irradiated dTCTP-depleted S2 cells compared with irradiated control cells ( Supplementary Fig. S7 ). Further, the kinetics of H2Av phosphorylation in dTCTP EY/h59 mutants showed that both the gross intensity of γ-H2Av stained wing disc and the number of γ-H2Av-positive cells are significantly reduced compared with wild-type ( Fig. 7d,e ). dTCTP directly modulates ATM kinase activity Since dTCTP directly binds to dATM, and phosphorylated H2Av level by dATM is reduced in dTCTP mutants, we inferred that dTCTP could be necessary for promoting dATM kinase activity through direct binding. To test this hypothesis, we assayed dATM kinase activity in vitro. First, we checked whether H2Av is used as a substrate of dATM as in mammals [6] , [40] . 2X FLAG-dATM was immunoprecipitated from transfected S2 cells using anti-FLAG antibody, and used to measure its kinase activity on two kinds of recombinant H2Av substrates, wild-type H2Av and mutant H2Av ΔCT (H2Av without the C-terminal 15 aa containing the site for phosphorylation). The wild-type H2Av was phosphorylated by the immunoprecipitated dATM in vitro ( Fig. 8a bottom panel, Lanes 1 and 5), whereas H2Av ΔCT was not ( Fig. 8a , Lane 9), indicating that H2Av is a specific substrate for dATM. Next, we checked whether dTCTP itself can facilitate dATM kinase activity on H2Av. An addition of dTCTP to dATM increased the phosphorylation level of H2Av in a concentration-dependent manner ( Fig. 8a , bottom panel, Lanes 2–4). In contrast, the mutated dTCTP E12V protein did not increase the H2Av phosphorylation ( Fig. 8a , Lanes 6–8). These results indicate that dTCTP can enhance dATM kinase activity through direct interaction. 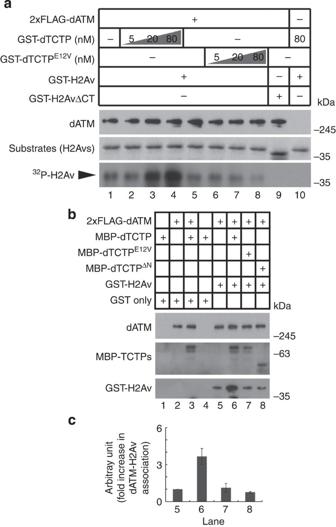Figure 8: dTCTP directly facilitates dATM kinase activity by enhancing enzyme–substrate association. (a)In vitrokinase assay. (Upper panel) western blot with anti-FLAG is used to show dATM protein loaded. (Middle panel) Coomassie blue staining of the substrate proteins loaded. The GST-fusion proteins (625 nM) were subjected to dATM phosphorylationin vitroand resolved by sodium dodecyl sulfate polyacrylamide gel electrophoresis followed by autoradiography. (bottom panel) Arrow points to phosphorylated H2Av. dATM enzyme activity is enhanced by wild-type dTCTP protein in a concentration-dependent manner (Lanes 2–4) but not by mutated dTCTP protein (E12V; Lanes 6–8). Lanes 9 and 10 are negative controls. A defective H2Av protein with a deletion in the phosphorylation site (H2AvΔCT) is not phosphorylated by dATM kinase (Lane 9). H2Av phosphorylation is not detected in the absence of dATM (Lane 10). (b,c) dTCTP facilitates binding of H2Av substrate to dATM (Lanes 5, 6). Immunopurified dATM (using agarose-bound anti-FLAG) was incubated with dTCTP protein variants, and then mixed with GST-H2Av or GST without ATP. Associated proteins were eluted and analysed using western blot with anti-FLAG, MBP or GST. Mutated dTCTP proteins do not increase H2Av binding affinity to dATM (Lanes 7, 8). (c) Quantification of H2Av binding affinity to dATM (normalized to Lane 5). Error bars are s.e.m. Performed in triplicate. Figure 8: dTCTP directly facilitates dATM kinase activity by enhancing enzyme–substrate association. ( a ) In vitro kinase assay. (Upper panel) western blot with anti-FLAG is used to show dATM protein loaded. (Middle panel) Coomassie blue staining of the substrate proteins loaded. The GST-fusion proteins (625 nM) were subjected to dATM phosphorylation in vitro and resolved by sodium dodecyl sulfate polyacrylamide gel electrophoresis followed by autoradiography. (bottom panel) Arrow points to phosphorylated H2Av. dATM enzyme activity is enhanced by wild-type dTCTP protein in a concentration-dependent manner (Lanes 2–4) but not by mutated dTCTP protein (E12V; Lanes 6–8). Lanes 9 and 10 are negative controls. A defective H2Av protein with a deletion in the phosphorylation site (H2Av ΔCT ) is not phosphorylated by dATM kinase (Lane 9). H2Av phosphorylation is not detected in the absence of dATM (Lane 10). ( b , c ) dTCTP facilitates binding of H2Av substrate to dATM (Lanes 5, 6). Immunopurified dATM (using agarose-bound anti-FLAG) was incubated with dTCTP protein variants, and then mixed with GST-H2Av or GST without ATP. Associated proteins were eluted and analysed using western blot with anti-FLAG, MBP or GST. Mutated dTCTP proteins do not increase H2Av binding affinity to dATM (Lanes 7, 8). ( c ) Quantification of H2Av binding affinity to dATM (normalized to Lane 5). Error bars are s.e.m. Performed in triplicate. Full size image To further define the mechanism of dTCTP stimulation on dATM kinase activity, we examined whether dTCTP affects the H2Av binding affinity to dATM in vitro . First, immunoprecipitated functional dATM proteins, which bind to dTCTP without substrates ( Fig. 8b , middle panel, Lane 1–4), were incubated with wild-type or mutant (E12V and ΔN) dTCTP proteins. This complex was then mixed with H2Av substrates for dATM kinase without ATP nucleotides. Western blot assay on these protein complexes showed that dATM alone can bind to H2Av substrates ( Fig. 8b , bottom panel, Lane 5). However, only wild-type dTCTP facilitates binding of H2Av to dATM by approximately threefold ( Fig. 8b , bottom panel and 8c; Lane 6) compared with no dTCTP or mutant dTCTP controls (Fig. 8c, Lanes 5–8). Earlier, we showed that the N-terminal region of dTCTP is necessary for promoting the binding between dTCTP and dATM ( Fig. 1b ). Failure of dTCTP ΔN to facilitate the binding of dATM to H2Av further supports the functional importance of this N-terminal domain. Altogether, these data suggest that dTCTP enhances the binding of dATM to H2Av substrates, thereby facilitating dATM kinase activity. TCTP has been implicated in a few events in cell nucleus, including transcription [41] , [42] , [43] . Recently, it has been reported that hTCTP in irradiated fibroblast participates in DSB repair through Ku translocation and colocalization with ATM. However, the nature of hTCTP interaction with ATM and its physiological significance in animals remains unknown [29] . Here, our in vivo studies, using Drosophila as an animal model, provide evidence that dTCTP is required for maintaining genome stability in mitotic cells of developing organs such as brain and wing discs, and endocycling cells of salivary glands. In response to induced DSBs, dTCTP mutants show reduced viability, abnormal array of ommatidia, increased DNA fragmentation, RDS (intra S checkpoint defect), G2/M checkpoint defect and increased apoptosis as a result of impaired checkpoints. Since these defects are similar in Drosophila atm mutants [14] , [15] , [38] , it is likely that the function of dTCTP for DSB repair is closely related with dATM. Indeed, both direct interaction and subcellular colocalization between them support this notion. Moreover, our genetic data and biochemical assays using dATM and its substrate (H2Av) illustrate that dTCTP directly facilitates dATM kinase activity by enhancing binding affinity of dATM to its substrate, providing a molecular basis for the relationship between TCTP and ATM that has not been studied before [29] . It is interesting to note that dATM is required for the formation of dTCTP foci but not vice versa . Hence, in the first place dTCTP may be recruited to nuclear foci depending on the presence of dATM. Once it is recruited to the DSB sites, dTCTP may function as a cofactor for positive modulation of dATM kinase activity, providing a mutually dependent mechanism for dATM activation. DSBs are repaired by one of the two major repair pathways: HR and NHEJ pathways. In HR, the activated ATM phosphorylates many proteins to facilitate DNA damage repair [44] . The MRN complex (a DSB sensor) is also required to activate and recruit ATM to DSB sites in HR pathway [5] , [45] . In NHEJ, DSBs are sensed by DNA-PKcs/Ku70/80 protein complex (DNA-PK holoenzyme) and repaired by Lig4 (ref. 9) [9] . Interestingly, a subset of HR-associated proteins such as MRN and ATM can interlink HR and NHEJ. For example, the MRN complex is partially involved in DSB end processing for NHEJ repair [9] . ATM also enhances the NHEJ process by phosphorylating the nuclease Artemis for DSB end processing [46] as well as Ku70/80 complex to enhance its binding affinity to DNA fragments [47] . Our genetic data show strong interactions between dTCTP and DDR genes for HR ( MRN , MDC , MCPH1 and his2Av ) and NHEJ ( MRN , lig4 and mus309 ( ku70 homologue)) ( Supplementary Fig. S6 and Supplementary Table S2 ). These results suggest that dTCTP can interlink HR and NHEJ in vivo . This idea is also consistent with a model recently proposed by Zhang et al . [29] that hTCTP interlinks the HR and NHEJ pathways. In this model, hTCTP promotes Ku70/80 complex translocation for NHEJ repair and forms a complex with ATM for HR repair, although its function in HR pathway has not been clearly defined. Collectively, these studies in human and fly strongly support that TCTP participates in both HR and NHEJ pathways to repair DSBs in eukaryotes. In addition to the fact that both Drosophila and hTCTP are involved in HR and NHEJ repair pathways, they have several other features in common. Reduced TCTP function results in increased chromosomal fragmentation by IR, IR sensitivity, RDS (G1/S-phase checkpoint defect) and G2 delay (G2/M checkpoint defect). TCTP also forms a complex with ATM in DSB sites and participate in NHEJ process for DNA repair by helping Ku translocation. However, there are also apparent differences between hTCTP and dTCTP. Unlike hTCTP, dTCTP protein level or stability is not affected by dATM or IR ( Supplementary Fig. S9 ). Importantly, dTCTP localization in the endocycling cells suggests that dTCTP is needed to repair not only induced DSBs but also naturally occurring DSBs in physiological condition. One of the most remarkable differences is shown in the phosphorylation level of H2A variant (γ-H2Av in fly and γ-H2AX in human) in the absence of TCTP. In irradiated human fibroblast, hTCTP depletion causes increases in DNA fragmentation and H2AX phosphorylation compared with the normal control. In contrast, reduction of dTCTP in dTCTP mutants leads to increased DNA fragmentation but reduced H2Av phosphorylation levels. Previous reports in Drosophila adult brain, mouse embryonic fibroblast and human osteoblastoma [11] , [40] , [48] have shown that H2Av/H2AX phosphorylation levels are considerably reduced in ATM-depleted conditions despite high DNA lesions, and our results ( Fig. 7 ) are on the same lines as these. Thus, our data support the hypothesis that TCTP directly enhances ATM kinase activity to repair DSBs, especially in the early DDR steps such as amplification of DSB signals through γ-H2AX formation by ATM. Our in vitro assay data ( Fig. 8 ) strongly support this concept. An intriguing question is how H2AX phosphorylation is increased in hTCTP-depleted fibroblasts, on the contrary to dTCTP- and ATM-depleted conditions. One possible explanation is that γ-H2AX might be formed by redundant functions of other kinases such as ATR or DNA-PK that can substitute the reduced ATM activity resulting from TCTP depletion. Such compensatory phosphorylation might be possible because both ATR and DNA-PK can phosphorylate H2AX to some extent against induced DSBs when ATM is depleted [40] , [48] , [49] . On the contrary, Drosophila atm 8 mutant shows little H2Av phosphorylation in response to induced DSBs [11] . Furthermore, Drosophila atr mutants show weak genetic interactions with ey>dTCTPi resulting in mildly enhanced eye phenotypes ( Supplementary Table S2 ). These may indicate that functional redundancy for dATM is restricted and that the mechanism to maintain genome stability in Drosophila is simpler than in human. It would be interesting to see whether TCTP proteins in other vertebrate systems function to control ATM activity as in Drosophila . Growing evidence suggests that mammalian ATMs are known to play additional roles in the cytoplasm, although the underlying mechanisms are not well understood [44] , [50] . Interestingly, recent studies suggested that human ATM regulates mTORC1 pathway either positively or negatively depending on the presence or absence of stresses [44] , [45] , [50] , [51] , [52] . Given that TCTP makes a complex with ATM and functions in both nucleus and cytoplasm, it could be possible that TCTP and ATM might share a function for modulating mTORC1 pathway. Fly genetics The w 1118 strain was used as the wild-type control. To obtain sufficient number of mutant animals for assaying dTCTP functions in DDR, we crossed dTCTP EY09182 / TM6b and dTCTP h59 / TM6b to create transheterozygous TCTP mutant, dTCTP EY09182 / dTCTP h59 . dTCTP h59 , dTCTP EY09182 , UAS-dTCTPi , UAS-dTCTP and UAS-dTCTP E12V were described elsewhere [25] . atm 3 , atm 6 and Df(3)PG4 were from Dr Shelagh D. Campbell (University of Alberta, Canada). The other strains were obtained from NIG-FLY, Vienna, and Bloomington stock centres. See Supplementary Information for more information. ImageJ (NIH) was used to quantify the number of ommatidia. Immunohistochemistry and fractionation of embryo extract Salivary and fat tissues were fixed in PLP fixative for 15 min at room temperature (RT). Primary antibodies were as follows: rabbit anti-dTCTP (1:300), mouse anti-tubulin (1:200, Sigma F2168) and rabbit anti-histone H2AvD pS137 (1:1,000, Rockland 600-401-914). Chromosomes were visualized with Vectashield (H-1200) with DAPI. For confocal analysis, Zeiss LSM 710 was used. For tissue staining, standard protocols were used [53] . For polytene chromosome staining [54] , third instar larvae were raised at 18 °C to obtain well-resolved band/interband pattern. Primary antibodies were used as follows: rabbit anti-dTCTP (1:300) and mouse anti-HP1 (1:50, DSHB C1A9-c). For S2 cell staining, primary antibodies were as follows: mouse anti-FLAG (1:200, Sigma F1804) and rabbit anti-c-MYC (1:250, Santa Cruz sc-789). To separate total embryo extract (0–20 h old, 38 mg) into cytosolic and nuclear protein fractions, NE-PER extraction kit was used (Thermo Scientific). Ten micrograms of each fraction was used for western blotting. Primary antibodies were as follows: rabbit anti-dTCTP (1:3,000), rabbit anti-dimethyl histone H3 (K4) (1:2000, Upstate 07–030), mouse anti-β-tubulin (1:2,000, DSHB E7-C). γ-H2Av and DAPI intensities were qualified using ZEN 2009 programme (Carl Zeiss). For western blot analysis in other tissues, four pairs of salivary glands and 30 pairs of wing discs were analysed for each genotype. Uncropped images of western blots are shown in Supplementary Fig. S10 . Assays for radiation sensitivity and genome stability For radiation sensitivity assay, 50 of second instar larvae were collected from grape juice plates and transferred into a food vial. Wandering third instar larvae were treated with the indicated doses of γ-radiation. The survival rate to adulthood of irradiated larvae was scored (the number of viable adult flies/the number of pupae). For chromosome instability assay in larval neuroblasts, third instar larvae were irradiated and rested for 1 h at RT. For larval neuroblast preparation, brains were dissected in 0.7% NaCl solution, incubated in 0.05 mM colchicine for 90–120 min, then transferred to a hypotonic solution (0.5% sodium citrate) for 10 min. Brains were fixed in 45% acetic acid for 1 min and in 60% acetic acid for 1 min, or in 45% acetic acid with 2% formaldehyde. To assay chromosome instability in adult wings, the wing hair phenotype caused by loss of heterozygosity of the multiple wing hair mutation was used as a marker [33] . Checkpoint and TUNEL assay To check G2/M checkpoint, 20–30 wandering third instar larvae, collected in a vial, were mock-or IR-treated and rested in a 25 °C incubator for 1 h. Dissected wing discs in phosphate-buffered saline (PBS) were fixed in PLP fixative for 20 min at RT, blocked and immunostained as previously described with some modifications. To label mitotic cells, a primary antibody against PH3 was used (1:200, Upstate 06–570). For determination of intra S checkpoint, brains were extirpated in M3 BPYE insect media and incubated for 10 min in the same medium containing 0.5 mg ml −1 BrdU (Sigma B8434, 10 mg ml −1 stock was prepared in 50% ethanol). These brains were fixed for 20 min in PBTx (PBS with 0.3% Triton X-100) containing 5% formaldehyde. After washing three times with PBTx, BrdU-labelled DNA was denatured with 3.0 N HCl for 30 min and neutralized with PBTx [37] . Primary antibody was mouse anti-BrdU (1:50, BD 347580). To assay cell death in wing discs, 25–30 wandering third instar larvae were collected in a food vial. Mock-or IR-treated larvae were rested in a 25 °C incubator for 4 h and then dissected in PBS. Wing discs attached on inside-out body cuticle were fixed in 4% formaldehyde in PBS with 0.1% triton X-100. TMR in situ cell death detection kit (Roche) was used for TUNEL staining. In vitro GST pull down MBP-tagged dTCTP and ATM 1006–1215 were cloned into pMAL-c2 vector (NEB). GST-tagged ATM and dTCTP variants were cloned into pGEX4T-1 (or 5X-1; GE Healthcare) vector. The primer sets used for PCR were listed in Supplementary Table S2 . GST-tagged and MBP-tagged proteins were expressed in E . coli Rosetta2 (BL21 derivatives; Novagen, Germany). IPTG induction was performed in 15 °C shaking incubator at 250 r.p.m. for 4 h. Recombinant proteins were extracted according to the resin manufacturer’s protocol (NEB and GE healthcare, USA). The extracted proteins were dialyzed in TBS buffer (20 mM Tris (pH 8.0), 150 mM NaCl) containing 20% glycerol and 1 mM DTT and stored at −20 °C before use. Five or ten micrograms of MBP fusion proteins were used as preys and the same amount of GST fusion proteins as baits. GST-binding resin was equilibrated in PDB (20 mM Tris·Cl, pH7.5), 150 mM NaCl, 0.5 mM EDTA, 10% Glycerol, 0.1% Triton X-100, 1 mM DTT, proteinase inhibitor cocktail (Roche). Protein complex was formed in PDB with 0.2% bovine serum albumin protein at 4 °C overnight and washed three times in PDB at RT. The samples were boiled in protein loading buffer at 94 °C for 5 min and loaded for western blotting. Primary antibody was a rabbit anti-MBP (1:10,000, NEB E8030S). co-IP To express dATM, Rad50, Mre11 and dTCTP in Drosophila S2 cell, these genes were PCR amplified from pAGW-ATM [55] , LP09268, LD08638 (DGRC, IN, USA), and pGEX-dTCTP plasmids, respectively. The primer sets used for PCR were listed in Supplementary Table S1 . The amplified PCR fragments were cloned into pAc5.1 vector (Invitrogen, USA) or its derivatives (pAc5.1-N′-tagged 2 × FLAG or 2 × c-MYC) using in-fusion cloning kit (Clontech, CA, USA). We used Stbl2 competent cell (Invitrogen) to clone atm cDNA. S2 cells were transfected using Effectene (Qiagen) according to the manufacturer's manual. An equal amount of plasmids was used for transfection. If the total amount of plasmid was different, pAc5.1 empty vector was added to obtain equal protein expression level. To perform Co-IP in S2 cell, cells were lysed on ice using a dunce homogenizer in cold IP buffer (50 mM HEPES (pH7.5), 50 mM KCl, 2 mM MgCl 2 , 1 mM EDTA (pH 8.0), 0.3% CHAPS, 1 mM DTT, 1 mM PMSF, proteinase inhibitor and phosphatase inhibitor cocktail (Roche)). Protein complexes were immunoprecipitated with rabbit anti-c-MYC (Abcam, Ab9106)-protein G agarose beads (Roche) or mouse anti-FLAG affinity gel (Sigma, A2220) at 4 °C for overnight. The immunocomplexes were washed three times with cold IP buffer at 4 °C. The samples were boiled in protein loading buffer at 94 °C for 5 min and loaded for western blotting. Primary antibodies were as follows: mouse anti-V5 (1:5,000, Invitrogen 46-0705), mouse anti-FLAG (1:2,000, Sigma F1804), mouse anti-c-MYC (1:2,000, sc47694) and rabbit anti-c-MYC (1:5,000, Abcam Ab9106). For Co-IP in pupal NEs, 200 white pupae were collected, frozen with liquid nitrogen (LN 2 ) and pulverized in LN 2 . Powdered homogenate was suspended in 2 ml of Buffer I (10 mM HEPES (pH7.6), 10 mM KCl, 5 mM MgCl 2 , 0.5 mM EDTA, 5% glycerol, 250 mM Sucrose, 1 mM DTT, 1 mM PMSF, proteinase inhibitor and phosphatase inhibitor cocktails (Roche)). After filtration of two layers of Miracloth (Calbiochem), the homogenate was centrifuged at 5,000 g for 20 min at 4 °C. The pellet was resuspended in Buffer II (10 mM HEPES (pH7.6), 0.1% NP-40, 100 mM KCl, 2 mM MgCl 2 , 0.05% deoxycholate, 0.5 mg ml −1 bovine serum albumin, 5% glycerol, 0.5 mM EDTA, 1 mM DTT, 1 mM PMSF, proteinase inhibitor and phosphatase inhibitor cocktails (Roche)) and solubilized by sonication. NE was obtained after centrifugation at 15,000 g for 1 h at 4 °C. After preclearing with protein G agarose beads, the NE was incubated with the appropriate antibody for overnight at 4 °C. The immunocomplexes were washed five times in Buffer II at 4 °C, and used for western blotting. For benzonase treatment, NE was incubated with 100 U ml −1 benzonase (EMD Millipore) for 1 h at RT. Primary antibodies were as follows: rat anti-dATM (1:500) and rat anti-dTCTP (1:3,000). In vitro kinase assay In vitro kinase assay was done as described with some modifications [40] , [56] , [57] . Briefly, about 1.8 × 10 8 of S2 cells were transiently transfected and harvested after 2 days induction. The cells were lysed using Dunce homogenizer and sonication in cold TGN buffer (50 mM Tris·Cl (pH 7.5), 150 mM NaCl, 1% tween 20, 0.3% NP-40) with proteinase and phosphatase inhibitors. The cleared lysate by centrifugation was incubated with mouse anti-FLAG affinity gel (Sigma, A2220) at 4 °C for 3 h. The beads were washed twice with TGN buffer, once with TGN with 0.5 M LiCl and twice with 1 × Kinase buffer (50 mM HEPES (pH 7.5), 50 mM KCl, 4 mM MnCl 2 , 6 mM MgCl 2 , 10% glycerol, 1 mM DTT, 10 μM ATP) containing phosphatase inhibitors. The beads were then incubated in a kinase mix (20 μl of kinase buffer, 625 nM substrate (GST-H2Av or GST-H2AvΔCT, 10 μCi of γ-[ 32 P]ATP, appropriate amount of GST-dTCTP) at 30 °C for 10 min. Rat anti-dATM antibody An atm fragment encoding amino acids 1006–1215 was amplified using first-strand cDNA made from embryonic total RNA, and cloned into pGEX vecctor. GST-tagged ATM 1006–1215 was used as antigens to immunize rat. MBP-tagged ATM 1006–1215 was used for affinity purification. Antibody production and purification were carried out by Abfrontier (Korea). Purified dATM antibody was suitable for immunoblotting (1:500) but not for immunohistochemistry. Statistics Statistical significance of all data was evaluated by the t -test (Microsoft Excel). Double-stranded RNA-mediated interference One microgram of PCR products with T7 promoter sequence ( pSK(−) RNAi, atm RNAi, or dTCTP RNAi; Supplementary Table S3 ) was used for production of double-stranded RNA (MEGAscript kit, Ambion). Bathing way was used for RNAi treatment [58] . S2 cells (purchased from DGRC, Indiana) were seeded in 12-well plates at 1 × 10 6 per well. To maximize target protein reduction by RNAi, S2 cells were treated twice with each 10 μg of double-stranded RNA on day 0 and day 3. How to cite this article : Hong, S.-T. and Choi, K.-W. TCTP directly regulates ATM activity to control genome stability and organ development in Drosophila melanogaster . Nat. Commun. 4:2986 doi: 10.1038/ncomms3986 (2013).